3D and 2D aromatic units behave like oil and water in the case of benzocarborane derivatives 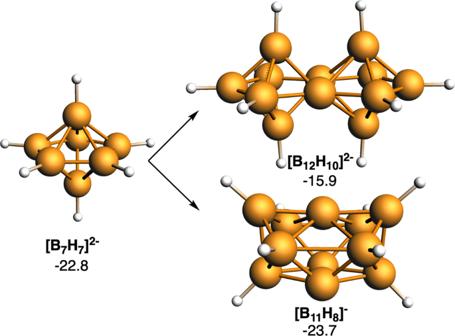Fig. 1: 3D/3D systems formed from [B7H7]2−. Computed NICS (in ppm) at the center of the five-membered ring of each cluster are enclosed. Boron atoms in orange and H atoms in white. A large number of 2D/2D and 3D/3D aromatic fusions that keep their aromaticity in the fused compounds have been synthesized. In addition, we have previously proven the electronic relationship between the 3D aromaticity of boron hydrides and the 2D aromaticity of PAHs. Here we report the possible existence of 3D/2D aromatic fusions that retain the whole aromaticity of the two units. Our conclusion is that such a 3D/2D aromatic combination is not possible due to the ineffective overlap between the π-MOs of the planar species and the n + 1 molecular orbitals in the aromatic cage that deter an effective electronic delocalization between the two fused units. We have also proven the necessary conditions for 3D/3D fusions to take place, and how aromaticity of each unit is decreased in 2D/2D and 3D/3D fusions. The two-dimensional (2D) aromaticity concept is widely accepted in all areas of science, and its most representative example is benzene. In 1978, Aihara [1] introduced the concept of 3D aromaticity, with the closo dodecaborate anion, [B 12 H 12 ] 2− , as its maximum exponent [2] . 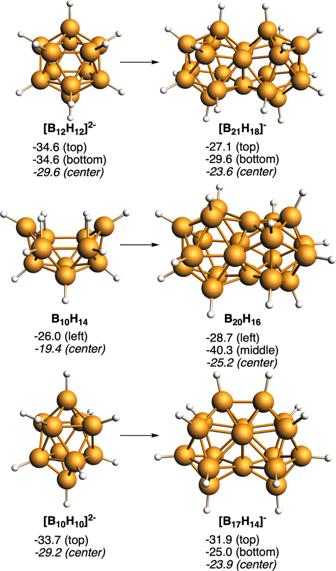Fig. 2: 3D/3D systems formed from [B12H12]2−, B10H14, and [B10H10]2−. Computed NICS (in ppm) at the center of different five- and four-membered rings and at the center of each cluster are enclosed. Boron atoms in orange and H atoms in white. Very recently, the concept of 3D aromaticity has been revisited. It has been established that a 3D aromatic compound must have a closed-shell electronic structure with at least triply degenerate molecular orbitals (MOs), extensive electron delocalization, and similar magnetic and electronic properties in the three xyz directions [3] . In 2014, an electronic relationship between 2D and 3D aromaticities was reported [4] , [5] , [6] , [7] . Conceptually, the 2D aromaticity can be easily extended with the fusion of two 2D aromatic units by sharing one edge. An example is the fusion of two benzenes sharing a common edge that gives rise to a new aromatic compound, naphthalene, and that following the same approach of sharing edges leads to polycyclic aromatic hydrocarbons (PAHs) [8] such as anthracene, pentacene, perylene, coronene, all the way to graphene, the wonder material of the twenty-first century [9] , [10] . PAHs are a class of chemicals that are found naturally in coal, crude oil, and gasoline [11] , but they are even found when burning any carbonaceous material [12] , [13] , or even when cooking meat and other foods at high temperature [14] , or in the interstellar space [15] . The ease with which they are produced is a consequence of the great stability that they have, largely due to the resonance property [16] . The high stability of 2D aromatic compounds is what favors their great diversity and the fact that they are found in key molecules for life such as hemoglobin, chlorophyll, and DNA bases. Indeed, there is an estimate that, according to PubChem, about two-thirds out of its 110 million structures of chemical compounds are fully or partially aromatic [17] . Just as there are so many experimental examples of PAHs resulting from the fusion of two 2D aromatic species, which we call 2D/2D for short, showing that the result is another aromatic 2D species, the question is: is the result of a fusion of two 3D/3D aromatic species another aromatic 3D species? And in line to the former one, we also raised the issue of whether it is possible that the fusion of two aromatic species, one 3D and the second 2D, a 3D/2D case, could result in a globally 3D/2D aromatic species. In this study, we will work as much as possible either with existing molecules or with their derivatives to provide a more consistent basis for the conclusions reached. Contrary to the 2D/2D fusion, there are very few examples available to demonstrate that the fusion of two 3D/3D aromatic entities leads to a molecule with 3D aromaticity. The reason for this is the lack of synthetic methods transferable from one process to another. However, two experimental examples have been found that will prove how the 3D/3D fusion results in a molecule with 3D aromaticity. These studies are based on boron hydride clusters, which are then expanded to hypothetical molecules with the same kind of structure based on existing 3D entities. It is interesting to note that in all known examples of fusions, whether 2D/2D or 3D/3D, the connecting atoms from the building blocks always had two outer electrons from a covalent bond, e.g., C–H or B–H. With this in mind, we have also explored units from polyanions derivatives of Zintl phase compounds [18] , [19] , e.g., [Sn 12 ] 2− , and fuse them together. The fusion results stress the importance that the connecting atom has one or two exocluster electrons, e.g. C in 2D aromatics or B in 3D aromatics have one electron, whereas Sn has two. We are aware of the recent synthesis of several fully π-conjugated macrocycles with strongly puckered or cage-type structures that have been considered 3D aromatic [20] , [21] . However, some authors consider that they are not truly 3D aromatic and rather they should be labeled as 2D-aromatic-in-3D [3] . Therefore, they cannot be used to analyze potential fused systems with 3D/3D aromaticity. Regarding the question whether the fusion of two entities, a 3D aromatic entity and a 2D aromatic entity, the 3D/2D case, results in a molecule with 3D/2D aromaticity, we will rely on experimental cases which have led to the fusion and demonstrate that in these circumstances the 3D entity retains its aromaticity but the 2D entity loses it. These examples have subsequently been extended to similar but hypothetical molecules that have corroborated these conclusions. 3D/3D fusions In 2014, we published that the electronic equivalent of benzene in boron hydrides was not [B 12 H 12 ] 2− but [B 7 H 7 ] 2− , i.e., both C 6 H 6 and [B 7 H 7 ] 2− share the same number of valence electrons [5] . Therefore, when fusing two benzene building blocks to give a naphthalene, the electronic equivalent in boron hydrides was [B 12 H 10 ] 2− , where two closo -B 7 units share an edge. This compound has not been synthesized but would most likely be stable if there were a pathway for its synthesis, as evidenced by its aromaticity, evaluated through the magnetic-based aromaticity criterion nucleus-independent chemical shift [4] , [5] , [6] , [22] , [23] (NICS—it is considered that the more negative the NICS value of a ring or cage, the higher its aromaticity—Fig. 1 ). Nonetheless, not in all cases more aromatic is related to more stable, as recently also proven by ourselves in related compounds [23] . If we stick only to the fusion of two [B 7 H 7 ] 2− units, there would be another closo alternative, which would be to share a face instead of an edge leading to [B 11 H 8 ] − . The pioneering work of Jemmis and other scientists [24] on a unified rule for predicting and systematizing structures of macropolyhedral boranes has really helped us in our analysis. As can be seen from the NICS shown in Fig. 1 , this second option would give rise to a species with a slightly more accentuated aromaticity than the previous one. [B 11 H 8 ] − has neither been synthesized, but its higher aromaticity seems to suggest that sharing a face provides more stability than sharing an edge. It is worth noting that [B 11 H 8 ] − with m = 2 and n = 11 and [B 12 H 10 ] 2- with m = 2 and n = 12 follow Jemmis’ mno rule of stability for fused boranes. According to this rule, the number of skeletal electron pairs required for a condensed polyhedral borane, carborane, heteroborane, metallaborane, or metallocene cluster to be aromatic is given by m + n + o , where m = number of sub-clusters, n = number of vertices, and o = number of single-vertex shared condensations [24] , [25] . Fig. 1: 3D/3D systems formed from [B 7 H 7 ] 2− . Computed NICS (in ppm) at the center of the five-membered ring of each cluster are enclosed. Boron atoms in orange and H atoms in white. Full size image These examples are at present imaginary, but are there any synthesized examples that demonstrate the fusion of 3D geometries? The answer is yes. In 2007, Bernhardt, Willner, and coworkers reported the elegant synthesis of [B 21 H 18 ] − from closo -[B 10 H 10 ] 2− to fac -[B 20 H 18 ] 2− to closo -[B 21 H 18 ] − , that they named a face-fused diicosahedral borate ion [26] . Earlier, in 1963, two separate groups, those of Lipscomb and Muetterties [27] , [28] , [29] , both using B 10 H 14 as starting reagent but with distinct synthetic strategies succeeded in synthesizing, isolating, and characterizing B 20 H 16 . Its structure, known by single-crystal determination, is consequence of the B 10 H 14 boat shape by facing two B 10 H 14 decks one rotated 90° so as to occupy the minimum volume. Do they share an edge or face? Of the two examples, the closo -[B 21 H 18 ] − shares one face, three boron atoms producing a global [(BH) 9 B 3 (BH) 9 ] − , and the B 20 H 16 can be interpreted as two [B 8 H 8 ] units joined by a B 4 diamond butterfly entity, producing a global [(BH) 8 B 4 (BH) 8 ]. Fig. 2 encloses the geometries of these fused compounds and their parent units. In addition, we have also proven the aromaticity, and thus its possible synthetic viability, of [B 17 H 14 ] − , which would be the result of the fusion of two archetypical species [B 10 H 10 ] 2− . It should be noted that the fusion of two [B 10 H 10 ] 2− building blocks involves connecting the two apical boron atoms, which are characterized by maintaining their exocluster B–H bonds. This link is also seen later with Sn. And with the aim of completeness, two other boron clusters but based on carboranes, i.e., CB 20 H 18 and [C 2 B 19 H 18 ] + , have been also analyzed. These are the fusion products of their also aromatic fusing components, [CB 11 H 12 ] − and C 2 B 10 H 12 , respectively (Fig. 3 ), and were previously proposed by Jemmis et al. [30] , who analyzed their isomerization energies and aromaticity. Here, we have focused only on the isomers in which the C atoms are located on the sharing triangular face derived from either [CB 11 H 12 ] − or C 2 B 10 H 12 [30] . We recently reported that the negative NICS values in [B 12 H 12 ] 2− and C 2 B 10 H 12 are the result of intense diatropic ring currents inside the cage [23] . Fig. 2: 3D/3D systems formed from [B 12 H 12 ] 2− , B 10 H 14 , and [B 10 H 10 ] 2− . Computed NICS (in ppm) at the center of different five- and four-membered rings and at the center of each cluster are enclosed. Boron atoms in orange and H atoms in white. Full size image Fig. 3: 3D/3D systems formed from [CB 11 H 12 ] − and C 2 B 10 H 12 . Computed NICS (in ppm) at the center of different five-membered rings and at the center of each cluster are enclosed. Boron atoms in orange, C atoms in gray, and H atoms in white. Full size image Finally, sandwich metallabis(dicarbollide) compounds (e.g., [Co(C 2 B 9 H 11 ) 2 ] − ) can be considered the result of the fusion between two nido -[C 2 B 9 H 12 ] − cages through a transition metal. In a recent work [23] , we showed that such metallabis(dicarbollide) species display global aromaticity with strong diatropic ring currents inside the two cages. All these boranes and carboranes obey the mno rule: [B 21 H 18 ] − ( m = 2, n = 21); B 20 H 16 ( m = 2, n = 20); [B 17 H 14 ] − ( m = 2, n = 17); [C 2 B 19 H 18 ] + and C 2 B 10 H 12 ( m = 2, n = 21); and [Co(C 2 B 9 H 11 ) 2 ] − ( m = 2, n = 23, o = 1) [24] . Both synthesized closo -[B 21 H 18 ] − and closo -B 20 H 16 are definitely aromatic as are their fusing components, [B 12 H 12 ] 2− , and B 10 H 14 , respectively. In fact, closo -B 20 H 16 with 22 skeletal electron pairs is aromatic and stable according to Jemmis’ mno rule. Remarkable are the connecting elements in fused aromatic hydrocarbons and aromatic closo boron hydrides, e.g., C 2 in naphthalene, (CH) 4 C 2 (CH) 4 and B 3 in [(BH) 9 B 3 (BH) 9 ] − , and B 4 in [(BH) 8 B 4 (BH) 8 ]. The connecting elements do not have any exocluster or exoring substituent when actually their parent components did have one or more exocluster substituents. The issue of the connecting elements is very relevant. For our purposes aimed at demonstrating the global aromaticity of fused 3D aromatic systems, we focus on merging components whose polyhedron is the icosahedron and the bicapped square antiprism. We have remarked that the connecting elements have no substituents outside the ring or cluster. Extending this idea to the elements with lone pairs means that the connecting elements have no electron pairs outside the cluster. In the case of the made [Sn 12 ] 2− (see ref. [31] ), a closo species with the same number of cluster electrons as [B 12 H 12 ] 2− , can be considered [32] . In the same way that the fusion of two [B 12 H 12 ] 2− gives rise to closo -[B 21 H 18 ] − one might think that the fusion of two [Sn 12 ] 2− would give rise to a [Sn 21 ] − . But that cannot be the case because of the electronic nakedness of the connecting elements. The electronically equivalent compound to closo -[B 21 H 18 ] − following the mno rule would be [Sn 21 ] 2+ , shown in Fig. 4 . Both compounds closo -[B 21 H 18 ] − and closo -[Sn 21 ] 2+ , resulting from 3D/3D fusions, are global aromatic and the same happens with closo -[Sn 17 ] 2+ , which arises from outstandingly aromatic closo -[Sn 10 ] 2− (Fig. 4 ), and that can be considered the equivalent to [B 17 H 14 ] − and its fusing [B 10 H 10 ] 2− unit, respectively (Fig. 2 ), sharing not only the same number of valence electrons but also their aromatic character. Remarkable is that the fused entities display considerably lower NICS values than their corresponding building blocks. Concern could here arise about the absolute interpretation of the NICS values for such heavy atoms like Sn, although it has been recently shown by Foroutan-Nejad et al. that the use of NICS is especially problematic when involving metals with half-filled shells, causing strong local paramagnetic currents. This is not our case, therefore its use in our closed-shell Sn clusters is most probably legitimate [33] , [34] . However, despite the relatively low negative NICS values found for fused Sn clusters as compared to those of borane clusters, the number of delocalized electrons per B or Sn atom obtained using QTAIM theory [35] , [36] of the series of Sn clusters and that of [B 10 H 10 ] 2− is very similar (Supplementary Fig. 2 ), thus supporting the aromatic character of both species. Moreover, there is a trend observed in all the reported fusions that is consistent with the aromaticity of fused moieties. The latter have always less negative NICS values than the building blocks. We attribute this reduction in the absolute value of NICS, first, to the intrinsic reduction in the aromaticity due to the fusion and, second, to the coupling between the magnetic fields of the two building blocks in the fused moieties. We can see from the above discussed NICS that the aromaticity of the pairs [B 21 H 18 ] – /[B 12 H 12 ] 2− , [B 17 H 14 ] – /[B 10 H 10 ] 2− , CB 20 H 18 /[CB 11 H 12 ] 2− , and [C 2 B 19 H 18 ] + /C 2 B 10 H 12 is reduced to a similar extent from the monomer to the dimer. Then, if we consider CB 20 H 18 and [C 2 B 19 H 18 ] + [30] , in both cases the connecting elements have carbons, one and two, respectively, or in other words, four or eight electrons are incorporated into the cluster. This enables the charge of the fused species to be more positive. These compounds with the highest atomic electron participation in the cluster turn out to be the fused compounds with the largest decrease from the monomer to the fused cluster. According to this reasoning, what happens with the fused Sn compounds, where there are more connecting elements with a contribution of four electrons each and are larger? As might be expected, the loss of aromaticity is more significant in this case, for both [Sn 21 ] 2+ /[Sn 12 ] 2− and [Sn 17 ] 2+ /[Sn 10 ] 2− . This leads to the important conclusion that it is much more difficult to fuse aromatic units of heavier elements than of lighter elements. Fig. 4: 3D/3D systems formed from [Sn 12 ] 2− and [Sn 10 ] 2− . Computed NICS (in ppm) at the center of different five- and four-membered rings and at the center of each cluster are enclosed. Sn atoms in gray. Full size image To this point, we can state that, for certain types of fusion and electronic charge of the cluster, the fusion of two aromatic halves of light elements results in another aromatic fused species and this stability seems to decrease with increasing atomic weight and the existence of lone pairs in the fusing atom which entail more positive charges in the fusion product, a factor which seems to be destabilizing. On this basis, we have begun with the most advantageous possible situation; we have merged equal halves in shape, size, and composition. For example, two benzenes or two dodecaborates. However, what happens if we fuse two 3D aromatic units of different size? For such, we have attempted the fusion of closo -[B 10 H 10 ] 2− and [B 12 H 12 ] 2− to smaller [B 6 H 6 ] 2− to give [B 13 H 10 ] − and [B 15 H 12 ] [− [38] , respectively, in which both monomers share a 3-membered face (Fig. 5 ). From the geometries, we can observe that [B 13 H 10 ] − also involves connecting the two apical boron atoms, whereas when the difference of size of the two units is larger, like in [B 15 H 12 ] − , this connection disappears. This latter point agrees with the work by Jemmis et al. stating that a large polyhedral borane condenses preferentially with a smaller polyhedron owing to orbital compatibility [37] . Importantly, the reduction of the aromaticity of the smaller unit ([B 6 H 6 ] 2− ) with the fusion is larger (from −30.7 to −21.0/−19.2 ppm) than for either [B 10 H 10 ] 2− (from −29.2 to −25.3 ppm) or [B 12 H 12 ] 2− (from −29.6 to −24.1 ppm). Fig. 5: 3D/3D systems formed from the fusion of [B 6 H 6 ] 2− and [B 12 H 12 ] 2− or [B 10 H 10 ] 2− . Computed NICS (in ppm) at the center of different four- and five-membered rings and at the center of each cluster are enclosed. Boron atoms in orange, and H atoms in white. Full size image 3D/2D fusions And then, what happens if we fuse a 3D aromatic unit with a 2D unit, in which one unit is larger than the second one? To make this situation more propitious, we will make both starting halves visible in the final product. For this purpose, 1,2-C 2 B 10 H 12 will be used, in which there are two contiguous carbons that can participate in the formation of a 6-carbon ring, a “benzene”. Before studying this case, we would like to recall that [B 12 H 12 ] 2− represents the archetype of 3D aromaticity, as stated above, and that any compound that can be formally derived from it must, in principle, be less or at the most equally aromatic than the reference compound. It is remarkable that the extraordinary stability of [B 12 H 12 ] 2− forces 1,2-C 2 B 10 H 12 , albeit incorporating two carbon atoms, to adapt to the geometry and aromaticity of [B 12 H 12 ] 2− (see ref. [23] ). Therefore, the C···C distance in neutral derivatives of 1,2-C 2 B 10 H 12 that spans from 1.64 to 1.82 Å [38] , is far from the usual distances in organic compounds approaching the B···B distance in [B 12 H 12 ] 2− that is ~1.8 Å. Consequently, due to the unequal C–C distance there will be a conflict of stabilities between one aromatic entity ~1.4 Å in benzene and ~1.7 Å in 1,2-C 2 B 10 H 12 . As a result, it may be that the C···C distance reaches an intermediate distance while maintaining a global aromaticity or that only one of the two entities maintains aromaticity, and in this case which of the two? In principle, we could assume that the one that has more to lose is going to be the winner. The optimal example to be studied is the formal fusion of 1,2-C 2 B 10 H 12 and benzene. Fortunately, the compound was previously synthesized and is known as the benzocarborane for which different synthetic methods have been described based on either o -carborane or carboryne as starting reagents [21] , [39] , [40] . Benzocarborane can also be synthesized from a transition metal-catalyzed [2 + 2 + 2] cycloaddition [41] of carboryne and two acetylene molecules (Fig. 6a ) [42] . The name benzocarborane implies that there is a benzene (aromatic) attached to a carborane whose aromatic condition was not indicated. The situation, as we shall see, is quite the opposite. Therefore, benzocarborane and its derivatives (Fig. 6 ) and its isomers (Fig. 7 ) are very adequate to address the question whether the 3D/2D aromatic fusion is feasible. Not too many alternatives exist that would facilitate this study. If the 2D fragment is made of carbons, this requires or at least makes it more likely, that the 3D fragment also contains adjacent carbon atoms in the structure, and that both are aromatic. In this context, o -carborane, 1,2-C 2 B 10 H 12 is key to study the 3D/2D fusion [43] . In difference, fullerenes may look appealing but either do not have 3D spherical aromaticity [44] or, reminding the issue of the connecting elements described earlier, how would it be possible to fuse with another aromatic half without sacrificing (at least partially) the aromaticity of the fullerene? As can be inferred from the above, only two aromatic halves with an outer electron pair in the system, either a C–H or a lone pair, can be fused. It is worth noting that we are not discussing the aromaticity of a phenyl group linked to a carborane, [PhCB 11 H 11 ] − , as reported recently by Muñoz-Castro (in this case both moieties remain aromatic) [45] but of benzo- o -carborane with the carborane cage and benzene ring fused. Also importantly, Xie and coworkers succeeded in the synthesis and X-ray characterization of substituted carboranes, and proved that there is considerable bond length alternation in the benzene ring (164.8–133.8 pm) ruling out aromaticity [42] , [46] . Similar alternation bond lengths were proven by Wade and coworkers on pristine benzo- o -carborane (165.1–133.8 pm) [47] , in agreement with the ethyl derivative. Fig. 6: 3D + 2D formation. a [2 + 2 + 2] cycloaddition between o -carboryne and alkynes; b structures of fused carborane and PAHS. Full size image NICS values very close to zero or to positive values indicate non-aromaticity, thus the computed data concerning the 2D fragment in Fig. 7 confirms the Matteson and Hota’s title of their article about benzocarborane, “High stability but little aromatic character” [40] . The NICS value of the 2D fragment is in significant contrast to that of o -carborane, which is very negative, indicating that just as the 2D fragment is not very aromatic, the 3D fragment is strongly aromatic. Therefore, of the two fragments, one retains aromaticity while the other clearly loses it. The four benzocarborane isomers studied and presented in Fig. 7 show the same trend, but it is worth noting that the one with the C 4 B 2 group occupying para positions relative to the two carbons of the carborane (benzene BBp ) has the most negative NICS values. These results point out that the fusion of two halves, each one known to be clearly aromatic, both suitable for the 3D/2D investigation does not lead to a global aromatic compound, but instead one of the two halves loses its aromaticity while the second retains its aromaticity. In the benzocarborane, the carborane keeps its aromaticity, with NICS only slightly reduced (from −33.3 to −33.0 ppm in the center of B 4 C five-membered ring (5-MR) and from −27.3 to −26.8 ppm in the center of cluster), however, the fused benzene becomes nonaromatic (NICS reduced from −8.1 to −1.5 ppm) as expected from the fact that the 6-MR contains only four π-electrons. The same trend is observed when benzene is fused to bonds other than C–C (Fig. 7 ). And the same behavior applies to larger PAHs: naphthalene, anthracene, and phenanthrene, when fused to o -carborane (Fig. 8 ). The only ring that gives an opposite behavior is the terminal one of phenanthrene. The reason is the presence of a Clar π-sextet [48] , [49] on this ring (Fig. 6b ), at difference to either naphthalene or anthracene that cannot accommodate such π-sextet (bond lengths also support this observation, Supplementary Fig. 1 ). This is the reason why only this ring remains fully aromatic. Fig. 7: Fused systems between o -carborane C 2 B 10 H 12 and benzene. NICS (in ppm) and nomenclature of the different isomers (BBo states for BB bond next to CC, whereas BBp states for the BB bond at the opposite site to the CC bond). NICS for C 2 B 10 H 12 are −33.3 and −27.3 ppm for the center of the B 4 C ring and center of the cluster (values in italics), respectively, and −8.1 ppm for benzene (see also Supplementary Tables 1 and 2 ). Boron atoms in orange, C atoms in gray, and H atoms in white. Full size image Fig. 8: Fused systems between o -carborane C 2 B 10 H 12 and benzene, naphthalene, anthracene, and phenanthrene. NICS (in ppm) for the five-membered rings and center of the carborane and MCI (in au) for the PAHs with and without (in italics) the carborane being attached (see also Supplementary Tables 1 and 2 ). Boron atoms in orange, C atoms in gray, and H atoms in white. Larger MCI values indicate higher electron delocalization in the ring. Full size image The difficulty for this 3D/2D fusion can be assigned to the lack of overlap between the π-MOs of the PAH and those of the carborane. A model system built from the system benzene CC above, analyzed through a quantitative molecular orbital and energy decomposition analyses, has allowed to confirm the ineffective overlap ( Supplementary Discussion ). Finally, let us mention that the above conclusions on 3D/2D fusion also apply to the fused carborane and five-membered heterocycles previously synthesized in ref. [50] . One of the fundamental characteristics of Hückel’s 2D aromaticity is the large number of aromatic species derived from the fusion of two aromatic halves. We have named these as 2D/2D aromatic fusions. Prior to this work, few 3D/3D aromatic fusions had been explicitly described [29] , although some examples had been synthesized and have been demonstrated in this work to be global aromatics. It has therefore been shown that such fusions are possible by the union of two 3D aromatic halves. The difficulty or impossibility for 3D/2D fusions is also proven in this work. The main reason for non-having a 3D/2D aromatic species is the ineffective overlap between the π-MOs of the PAH and the n + 1 MOs in the cage that deter a higher electronic delocalization between the two fused units. Furthermore, it is proven that for 3D/3D fusions to take place, some conditions have to be fulfilled. The first and obvious one is that each of the halves to be merged must be aromatic. The halves to be fused must have a great similarity in the two-connecting atom distances, although in borane clusters, 3D units of different size favor fusion [37] . The participating elements in the fusion must have exocluster bonds, e.g., C–H, B–H in the starting half or lone pairs. These connecting elements will be distinct in the fused molecule from other participating elements and will not have exocluster bonds. To our understanding, these conditions appear to be necessary for fusions of aromatic species to give rise to a global aromatic, but may not be sufficient. It seems that it can be generalized that aromaticity decays with fusion, this is observed in all 2D/2D, 3D/3D, and 3D/2D cases, being in the latter case dramatic as the 2D aromaticity vanishes completely. It is worth noting that the aromaticity decays comparably from 2D to 2D/2D as from 3D to 3D/3D. Fusion is more feasible with elements of the second period, C and B, and probably as one moves down the periodic table the aromaticity decreases. This has been seen with Sn in period 5, although it is in the same group as C. To be a connecting element, the atom in question must have an exocluster or exoring electron pair, e.g., C–H, B–H or Sn. The existence of lone pairs, however, leads to cationic charged species which can be potentially destabilizing. All calculations were performed with the Gaussian 09 package [51] by means of the B3LYP [52] , [53] , [54] hybrid density functional and the 6–311 + +G(d,p) basis set [55] . The geometry optimizations were carried out without symmetry constraints (Supplementary Data 1 ). Analytical Hessians were computed to characterize the optimized structures as minima (zero imaginary frequencies). Sn cluster have been computed by means of AMS 2021 software at ZORA-B3LYP-D3BJ/TZ2P level [56] , [57] . Aromaticity was evaluated by means of the nucleus-independent chemical shift (NICS) [4] , [5] , [6] , [22] , [23] , proposed by Schleyer and coworkers as a magnetic descriptor of aromaticity. NICS is defined as the negative value of the absolute shielding computed at a ring center or at some other point of the system. Rings with large negative NICS values are considered aromatic. NICS values were computed using the gauge-including atomic orbital method (GIAO) [58] . Multicenter indices (MCI) [59] , [60] , [61] and delocalization indices (DI) [35] , [36] were computed with the ESI-3D program using AIM partition of space [62] , [63] . 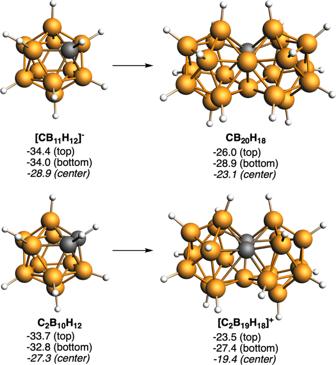Fig. 3: 3D/3D systems formed from [CB11H12]−and C2B10H12. Computed NICS (in ppm) at the center of different five-membered rings and at the center of each cluster are enclosed. Boron atoms in orange, C atoms in gray, and H atoms in white. 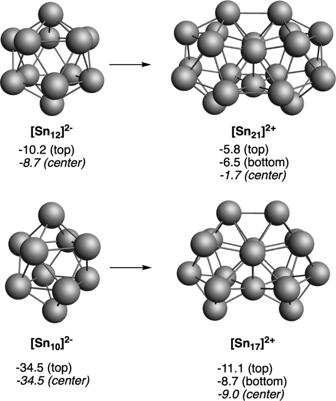Fig. 4: 3D/3D systems formed from [Sn12]2−and [Sn10]2−. Computed NICS (in ppm) at the center of different five- and four-membered rings and at the center of each cluster are enclosed. Sn atoms in gray. 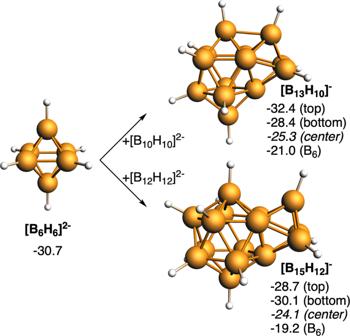Fig. 5: 3D/3D systems formed from the fusion of [B6H6]2−and [B12H12]2−or [B10H10]2−. Computed NICS (in ppm) at the center of different four- and five-membered rings and at the center of each cluster are enclosed. Boron atoms in orange, and H atoms in white. 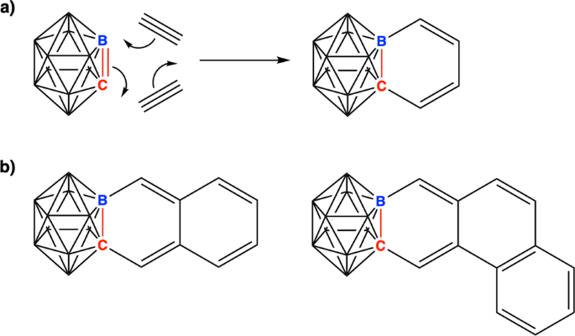Fig. 6: 3D + 2D formation. a[2 + 2 + 2] cycloaddition betweeno-carboryne and alkynes;bstructures of fused carborane and PAHS. 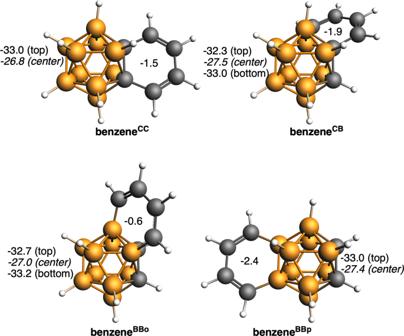Fig. 7: Fused systems betweeno-carborane C2B10H12and benzene. NICS (in ppm) and nomenclature of the different isomers (BBo states for BB bond next to CC, whereas BBp states for the BB bond at the opposite site to the CC bond). NICS for C2B10H12are −33.3 and −27.3 ppm for the center of the B4C ring and center of the cluster (values in italics), respectively, and −8.1 ppm for benzene (see also Supplementary Tables1and2). Boron atoms in orange, C atoms in gray, and H atoms in white. 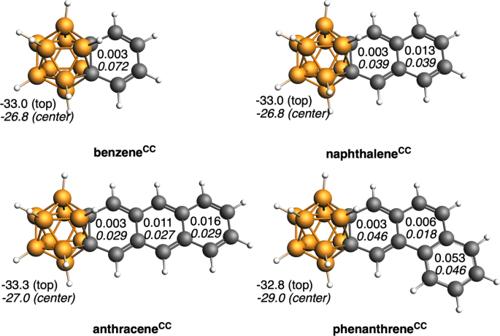Fig. 8: Fused systems betweeno-carborane C2B10H12and benzene, naphthalene, anthracene, and phenanthrene. NICS (in ppm) for the five-membered rings and center of the carborane and MCI (in au) for the PAHs with and without (in italics) the carborane being attached (see also Supplementary Tables1and2). Boron atoms in orange, C atoms in gray, and H atoms in white. Larger MCI values indicate higher electron delocalization in the ring. For completeness, the aromaticity of the enclosed systems has been further confirmed by means of bond length alternation (BLA) measures (Supplementary Table 3 ).